A half-metallic A- and B-site-ordered quadruple perovskite oxide CaCu3Fe2Re2O12with large magnetization and a high transition temperature Strong correlation between spins and conduction electrons is key in spintronic materials and devices. A few ferro- or ferrimagnetic transition metal oxides such as La 1− x Sr x MnO 3 , Fe 3 O 4 , CrO 2 and Sr 2 FeMoO 6 have spin-polarized conduction electrons at room temperature, but it is difficult to find other spin-polarized oxides with high Curie temperatures (well above room temperature) and large magnetizations for spintronics applications. Here we show that an A- and B-site-ordered quadruple perovskite oxide, CaCu 3 Fe 2 Re 2 O 12 , has spin-polarized conduction electrons and is ferrimagnetic up to 560 K. The couplings between the three magnetic cations lead to the high Curie temperature, a large saturation magnetization of 8.7 μ B and a half-metallic electronic structure, in which only minority-spin bands cross the Fermi level, producing highly spin-polarized conduction electrons. Spin polarization is confirmed by an observed low-field magnetoresistance effect in a polycrystalline sample. Optimization of CaCu 3 Fe 2 Re 2 O 12 and related quadruple perovskite phases is expected to produce a new family of useful spintronic materials. Materials with spin-polarized conduction electrons are of considerable interest in magnetic and electronic materials’ research and for technological applications such as spin-polarized field emission and spin-polarized tunnelling devices [1] . The Heusler alloy NiMnSb was the first predicted half-metallic ferromagnet [2] , and the oxides CrO 2 (refs 3 , 4 ) and Fe 3 O 4 (refs 5 , 6 ) also have half-metallic electronic structures and were intensively investigated. Discovery of colossal magnetoresistances in perovskite (for example, La 1− x Sr x MnO 3 ) and pyrochlore (for example, Tl 2 Mn 2 O 7 ) manganese oxides cast further light on the importance of strong correlations of spins and electrons in half-metallic transition metal oxides [7] , [8] , [9] , [10] . In the hole-doped Mott insulator La 1− x Sr x MnO 3 , double exchange between Mn 3+ and Mn 4+ mediated by the itinerant holes results in ferromagnetic spin ordering [11] , [12] , [13] and a half-metallic electronic band structure [14] , [15] . The high spin polarization of conduction electrons enabled novel spintronic devices to be developed, for example, a spin-dependent tunnelling trilayer structure where tunnelling conduction depends on the spin polarization of two electrodes [16] , [17] , [18] . This leads to large tunnelling magnetoresistance (TMR) in a low magnetic field, which can be exploited in high-performance magnetic sensors and extremely high-density memories. Although a large TMR was observed in such trilayer devices at low temperatures, the TMR ratio became small at room temperature because the degree of spin polarization decreases significantly near the magnetic transition temperature. Materials that have highly spin-polarized conduction electrons at room temperature and hence a magnetic transition temperature well above 300 K are therefore very desirable for further spintronic developments. Transition metal oxides with an ordered double-perovskite structure A 2 BB′O 6 , where the transition metal ions B and B′ are arranged alternately in a rock-salt manner [19] , [20] , [21] , are useful materials for spintronic applications [22] , [23] . An important example is Sr 2 FeMoO 6 , which is half-metallic and shows substantial TMR at room temperature [24] . The B-site Fe 3+ (3 d 5 , S =5/2) and the B′-site Mo 5+ (4 d 1 , S =1/2) spins couple antiferromagnetically, leading to ferrimagnetism. Below the magnetic transition temperature ( T c =410 K) only the minority-spin bands, which mainly consist of Fe 3 d t 2g and Mo 4 d t 2g orbitals hybridized with O 2 p orbitals, cross the Fermi level ( E F ), producing spin-polarized conduction electrons. A recent Monte Carlo study of Sr 2 FeMoO 6 showed that the electron spin polarization is proportional to the core spin magnetization and depends on temperature and disorder [25] , [26] . We have explored a strategy for enhancing spintronic properties relative to double perovskites by introducing further magnetic cations that can participate in a 1:3 order at the A sites, leading to the discovery of a new A- and B-site ordered quadruple perovskite oxide with large magnetization and a high magnetic ordering temperature. The A- and B-site-ordered quadruple perovskite-structure oxide is derived from the A-site-ordered perovskite with general formula AA′ 3 B 4 O 12 , which consists of a framework with heavily in-phase tilted BO 6 octahedra and A′O 4 squares [21] . Unlike the A site in the basic ABO 3 perovskites, which is usually occupied by alkali-metal, alkaline-earth or rare-earth cations, the A′ site in AA′ 3 B 4 O 12 can accommodate transition metal ions. The introduction of A′–A′ and A′–B magnetic interactions in addition to B – B couplings gives rise to a variety of intriguing properties [27] , [28] . For example, in CaCu 3 B 4 O 12 materials with A′=Cu 2+ and nonmagnetic ions at the B site, the A′–A′ interaction is ferromagnetic for B=Ge and Sn but antiferromagnetic for B=Ti [29] , [30] . When magnetic species like Mn are introduced into the B sites, the A′(Cu) – B(Mn) antiferromagnetic interaction becomes dominant and ferrimagnetism is observed in ACu 3 Mn 4 O 12 for A=Ca, La and Bi [31] , [32] , [33] . In the present study we prepared an AA′ 3 B 2 B′ 2 O 12 A- and B-site-ordered quadruple perovskite oxide to explore whether the advantages of an A-site-ordered AA′ 3 B 4 O 12 perovskite and an A 2 BB′O 6 double perovskite can be combined. The AA′ 3 B 2 B′ 2 O 12 crystal structure consists of 1:3 ordered A and A′ cations and rock-salt-ordered B and B′ cations ( Fig. 1 ). A few compounds with this structure type were already known, but none are half-metallic. CaCu 3 Cr 2 Sb 2 O 12 and CaCu 3 Fe 2 Sb 2 O 12 have nonmagnetic Sb 5+ ions at the B′ site so antiferromagnetic A′(Cu 2+ )–B(Cr 3+ /Fe 3+ ) interactions are dominant and these materials are ferrimagnetic insulators with T c ’s of 160 and 170 K, respectively [34] , [35] . In contrast, CaCu 3 Cr 2 Ru 2 O 12 is metallic but shows Pauli-paramagnetic behaviour [36] . 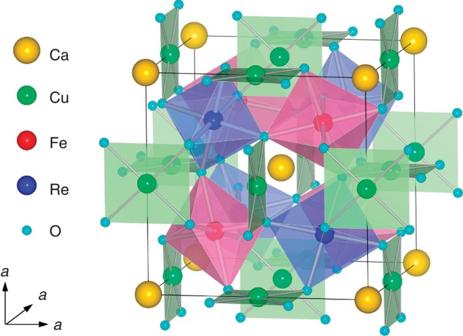Figure 1: Crystal structure of the A- and B-site-ordered quadruple perovskite CaCu3Fe2Re2O12. Ca and Cu ions are ordered in a 1:3 ratio at the A sites and Fe and Re ions are ordered in a rock-salt-type arrangement on the B sites of the ABO3perovskite structure, resulting in a framework of CuO4square units and heavily tilted FeO6and ReO6octahedra. We have explored other materials in which both B-site cations have potentially mobile d electrons that may give rise to half-metallic ground states for spintronic applications, resulting in the discovery of CaCu 3 Fe 2 Re 2 O 12 , which has highly spin-polarized conduction electrons and is ferrimagnetic with a large magnetization up to T c =560 K. Figure 1: Crystal structure of the A- and B-site-ordered quadruple perovskite CaCu 3 Fe 2 Re 2 O 12 . Ca and Cu ions are ordered in a 1:3 ratio at the A sites and Fe and Re ions are ordered in a rock-salt-type arrangement on the B sites of the ABO 3 perovskite structure, resulting in a framework of CuO 4 square units and heavily tilted FeO 6 and ReO 6 octahedra. Full size image Crystal structure of CaCu 3 Fe 2 Re 2 O 12 A polycrystalline sample of CaCu 3 Fe 2 Re 2 O 12 was obtained by synthesis under a high pressure (10 GPa) and high temperature (1400 K), as described in Methods. The sample was confirmed from synchrotron X-ray diffraction (SXRD) to be single phase and crystallized in a cubic 2 a 0 × 2 a 0 × 2 a 0 A-site-ordered perovskite structure. ( a 0 ≈4 Å is the lattice constant of a simple perovskite ABO 3 .) Observation of ( h k l ) reflections with odd h , k , l values evidences rock-salt-type ordering of the B and B′ cations with Pn space group symmetry. These B-site-ordering superstructure SXRD peaks were found to be broad compared with the fundamental reflections (which have even values of h+k+l ). This shows that the B-site Fe/Re ordering does not extend over the full scale of the crystallites, and the Fe/Re ordering coherence length was estimated to be ≈140 nm (190 unit cell lengths) from modelling the broadening with a Scherrer term in the Rietveld fit. No apparent oxygen off-stoichiometry was observed and the oxygen site occupancy was set to be unity in the refinement. The high X-ray scattering contrast between Fe and Re enabled precise B-site occupancies to be determined, from which a small inversion disorder of 6.2(1)% was found. The SXRD structure refinement thus confirms that CaCu 3 Fe 2 Re 2 O 12 has the quadruple perovskite structure with well-ordered A- and B-site cations. The fit is shown in Fig. 2 and the refined structure parameters and bond distances are listed in Tables 1 and 2 . 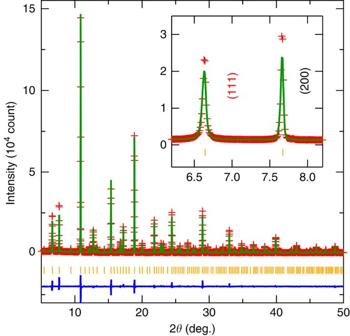Figure 2: Fit to the SXRD pattern of CaCu3Fe2Re2O12at room temperature. Observed intensity points (crosses), the calculated profile (full curve) and the difference between the observed and calculated intensities (offset curve below) are shown. The ticks indicate the Bragg peak positions. The inset shows an expanded view of the low-angle (1 1 1) and (2 0 0) diffraction peaks from which additional Scherrer broadening of (1 1 1) due to limited-range coherence of Fe/Re cation order is seen. Figure 2: Fit to the SXRD pattern of CaCu 3 Fe 2 Re 2 O 12 at room temperature. Observed intensity points (crosses), the calculated profile (full curve) and the difference between the observed and calculated intensities (offset curve below) are shown. The ticks indicate the Bragg peak positions. The inset shows an expanded view of the low-angle (1 1 1) and (2 0 0) diffraction peaks from which additional Scherrer broadening of (1 1 1) due to limited-range coherence of Fe/Re cation order is seen. Full size image Table 1 Refined structure parameters of CaCu 3 Fe 2 Re 2 O 12 at room temperature. Full size table Table 2 M–O distances and BVS calculated for CaCu 3 Fe 2 Re 2 O 12 from the structure analysis results in Table 1. Full size table Four of the 12 Cu–O distances are short, 2.006(5) Å, revealing the square-planar coordination of oxygen around the A′ site, and the resulting distortion leads to heavy tilting of the FeO 6 and ReO 6 octahedra. The cation valence states estimated from the observed cation–oxygen bond distances by a bond valence sum method [37] are shown in Table 2 . The bond valence sum values are very close to the formal values in the formula Ca 2+ Cu 2+ 3 Fe 3+ 2 Re 5+ 2 O 12 . The charge difference between Fe 3+ and Re 5+ results in the high degree of rock-salt-type cation ordering at the B/B′ sites. The same formal charge distribution was observed in CaCu 3 Fe 2 Sb 2 O 12 (ref. 35 ) and in the low-temperature charge-ordered phase of CaCu 3 Fe 4 O 12 where B-site charge disproportionation below 210 K stabilizes the Ca 2+ Cu 2+ 3 Fe 3+ 2 Fe 5+ 2 O 12 configuration [38] . Magnetic properties of CaCu 3 Fe 2 Re 2 O 12 Magnetization measurements for CaCu 3 Fe 2 Re 2 O 12 are shown in Fig. 3 . A high-temperature Curie transition is observed at T c =560 K, below which a large magnetization develops with a saturation value of 8.7 μ B per formula unit (f.u.) at 5 K. Spins from the Cu 2+ (3 d 9 , S =1/2), Fe 3+ (3 d 5 , S =5/2) and Re 5+ (5 d 2 , S =1) ions all contribute to the net magnetization of CaCu 3 Fe 2 Re 2 O 12 . Ferromagnetic Cu 2+ (↑)–Fe 3+ (↑)–Re 5+ (↑) alignment of the spins gives an ideal saturated magnetization of 17 μ B f.u. −1 , neglecting orbital contributions, while the collinear ferrimagnetic combinations Cu 2+ (↓)–Fe 3+ (↑)–Re 5+ (↑), Cu 2+ (↑)–Fe 3+ (↑)–Re 5+ (↓) or Cu 2+ (↑)–Fe 3+ (↓)–Re 5+ (↑) are respectively predicted to give 11, 9 or 3 μ B f.u. −1 . The observed saturated magnetization of 8.7 μ B f.u. −1 is thus close to the ferrimagnetic Cu 2+ (↑)–Fe 3+ (↑)–Re 5+ (↓) value. 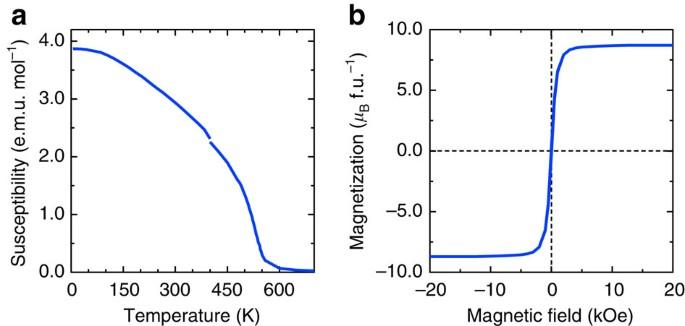Figure 3: Magnetic properties of CaCu3Fe2Re2O12. (a) Temperature dependence of magnetic susceptibility measured under an external field of 10 kOe, with the magnetic transition observed at 560 K. (b) Magnetization-field measurements at 5 K, revealing a large saturated magnetization of 8.7μBf.u.−1. The low-field region is expanded inFig. 7b. Figure 3: Magnetic properties of CaCu 3 Fe 2 Re 2 O 12 . ( a ) Temperature dependence of magnetic susceptibility measured under an external field of 10 kOe, with the magnetic transition observed at 560 K. ( b ) Magnetization-field measurements at 5 K, revealing a large saturated magnetization of 8.7 μ B f.u. −1 . The low-field region is expanded in Fig. 7b . Full size image Ferromagnetic coupling between Cu 2+ and Fe 3+ moments was confirmed by magnetic circular dichroism (MCD) intensities from X-ray absorption spectroscopy (XAS) measurements at 15 K, as shown in Fig. 4 . The observed XAS spectrum near the Cu edge is similar to that of square-planar Cu 2+ in BiCu 3 Mn 4 O 12 (ref. 39 ), although satellite structures due to the charge-transfer screening process are seen in the present CaCu 3 Fe 2 Re 2 O 12 , and the Fe spectrum is similar to the typical Fe 3+ O 6 signal in LaFeO 3 (ref. 40 ). The L 3 -edge MCD intensities are negative for both Cu and Fe, and the L 2 -edge intensities are positive for both metals—the coincident signs at each edge demonstrate that the spins of the A′-site Cu 2+ and B-site Fe 3+ ions couple ferromagnetically. The magnetic moments obtained from the MCD intensities by using magneto-optical sum rules [41] , [42] are 0.86 μ B (spin part, 0.82 μ B ) for Cu and 4.17 μ B (spin part, 4.11 μ B ) for Fe, in reasonably good agreement with the expected moments for Cu 2+ ( S =1/2) and Fe 3+ ( S =5/2). Analysis of preliminary powder neutron diffraction also supports the spin ordering model, as shown in Supplementary Fig. 1 and Supplementary Table 1 . 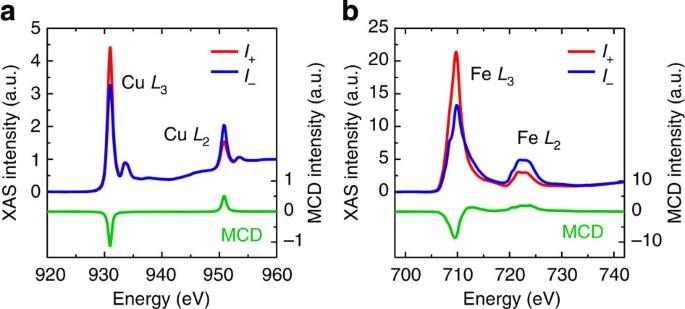Figure 4: XAS and MCD intensities of CaCu3Fe2Re2O12. (a) XAS and MCD intensities near the CuL3andL2-edges. (b) XAS and MCD intensities near the FeL3andL2-edges. Data were obtained at 15 K. The red and blue curves, respectively, represent XAS spectra measured with photon spins parallel (I+) and antiparallel (I−) to the magnetization direction of the sample, in which a static magnetic field of 19 kOe was applied. The MCD intensity was calculated as the difference between theI+andI−absorption spectra. The coincident signs of the Cu and Fe MCD intensities at eachL-edge show that their spins couple ferromagnetically. Figure 4: XAS and MCD intensities of CaCu 3 Fe 2 Re 2 O 12 . ( a ) XAS and MCD intensities near the Cu L 3 and L 2 -edges. ( b ) XAS and MCD intensities near the Fe L 3 and L 2 -edges. Data were obtained at 15 K. The red and blue curves, respectively, represent XAS spectra measured with photon spins parallel ( I + ) and antiparallel ( I − ) to the magnetization direction of the sample, in which a static magnetic field of 19 kOe was applied. The MCD intensity was calculated as the difference between the I + and I − absorption spectra. The coincident signs of the Cu and Fe MCD intensities at each L -edge show that their spins couple ferromagnetically. Full size image The ferrimagnetic spin structure of CaCu 3 Fe 2 Re 2 O 12 differs markedly from those of related cation-ordered perovskites, most notably in having ferromagnetic coupling between A′-site Cu 2+ and the dominant B-site Fe 3+ spins, as illustrated in Fig. 5 . The double-perovskite Ca 2 FeSbO 6 with nonmagnetic Sb 5+ ions at the B′ sites shows spin-glass behaviour at low temperatures due to geometric frustration of antiferromagnetic interactions within the tetrahedral B sublattice of Fe 3+ moments ( Fig. 5a ) [43] . Introducing Cu 2+ at the A′ site to give CaCu 3 Fe 2 Sb 2 O 12 relieves the spin frustration leading to ferrimagnetism below 170 K, but the Cu 2+ spins couple antiferromagnetically with the B-site Fe 3+ spins ( Fig. 5b ) [35] . This was confirmed by the MCD intensities of CaCu 3 Fe 2 Sb 2 O 12 , which are positive/negative at the Fe L 2 / L 3 -edges but negative/positive for Cu L 2 / L 3 -edges, in contrast to the spectra for CaCu 3 Fe 2 Re 2 O 12 shown in Fig. 4 . In charge-disproportionated CaCu 3 Fe 4 O 12 (CaCu 2+ 3 Fe 3+ 2 Fe 5+ 2 O 12 ), the Cu 2+ spins at the A′ site also couple antiferromagnetically with B-site Fe 3+ as well as with the B′-site Fe 5+ spins ( Fig. 5c ) [38] , [44] and the ferrimagnetic spin structure stabilized below 210 K is different to that of CaCu 3 Fe 2 Re 2 O 12 ( Fig. 5d ) regarding the B-site Fe 3+ spin direction. A strong A′(Cu 2+ )–B′(Re 5+ ) antiferromagnetic interaction in CaCu 3 Fe 2 Re 2 O 12 evidently outweighs the A′(Cu 2+ )–B(Fe 3+ ) interaction leading to ferromagnetic A′(Cu 2+ )–B(Fe 3+ ) spin alignment. 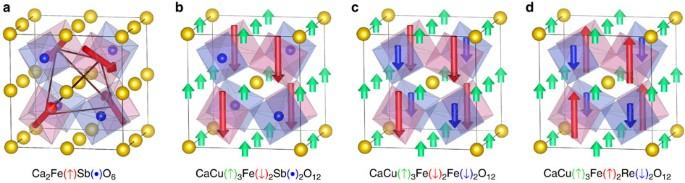Figure 5: Spin structures of perovskites with Fe3+ions at cation-ordered B sites. (a) The double-perovskite Ca2FeSbO6with a spin-glass transition temperature of 17 K. Order of antiferromagnetically interacting Fe3+spins is frustrated due to the tetrahedral geometry of the B sublattice. (b) A- and B-site-ordered quadruple perovskite CaCu3Fe2Sb2O12with nonmagnetic Sb5+at the B′ site andTc=170 K. A′-site Cu2+spins couple antiferromagnetically with the B-site Fe3+spins. (c) Charge-disproportionated CaCu3Fe4O12withTc=210 K, where A′-site Cu2+spins couple antiferromagnetically with the B-site Fe3+and B′-site Fe5+spins. (d) CaCu3Fe2Re2O12where A′-site Cu2+spins couple ferromagnetically with the B-site Fe3+and antiferromagnetically with the B′-site Re5+spins, leading to a highTcof 560 K and a large magnetization of 8.7μBf.u.−1. Figure 5: Spin structures of perovskites with Fe 3+ ions at cation-ordered B sites. ( a ) The double-perovskite Ca 2 FeSbO 6 with a spin-glass transition temperature of 17 K. Order of antiferromagnetically interacting Fe 3+ spins is frustrated due to the tetrahedral geometry of the B sublattice. ( b ) A- and B-site-ordered quadruple perovskite CaCu 3 Fe 2 Sb 2 O 12 with nonmagnetic Sb 5+ at the B′ site and T c =170 K. A′-site Cu 2+ spins couple antiferromagnetically with the B-site Fe 3+ spins. ( c ) Charge-disproportionated CaCu 3 Fe 4 O 12 with T c =210 K, where A′-site Cu 2+ spins couple antiferromagnetically with the B-site Fe 3+ and B′-site Fe 5+ spins. ( d ) CaCu 3 Fe 2 Re 2 O 12 where A′-site Cu 2+ spins couple ferromagnetically with the B-site Fe 3+ and antiferromagnetically with the B′-site Re 5+ spins, leading to a high T c of 560 K and a large magnetization of 8.7 μ B f.u. −1 . Full size image The T c =560 K of CaCu 3 Fe 2 Re 2 O 12 is much greater than those of the materials shown in Fig. 5 or indeed of any 1:3 A-site-ordered perovskites reported to date. The very high Curie temperature of CaCu 3 Fe 2 Re 2 O 12 is indicative of strong antiferromagnetic B(Fe 3+ )–B′(Re 5+ ) coupling, as ferrimagnetic A 2 FeReO 6 double perovskites have comparable T c ’s (of 520, 400 and 300 K for A=Ca, Sr and Ba, respectively) [22] , [45] , [46] , [47] , [48] . It is notable that CaCu 3 Fe 2 Re 2 O 12 has a higher T c than Ca 2 FeReO 6 and a greater saturated magnetization (8.7 μ B f.u. −1 versus 4.7 μ B (double f.u.) −1 of Ca 2 FeReO 6 (ref. 49 )). A further difference is that CaCu 3 Fe 2 Re 2 O 12 is a soft ferrimagnet with a coercive field of ~100 Oe and so is well-suited to low-field switching in spintronic devices, whereas Ca 2 FeReO 6 is a hard magnetic material with a large coercivity of ≈10 kOe (refs 47 , 49 ). Magnetic anisotropy due to spin-orbit coupling of Re 5+ is strongly coupled to the monoclinically distorted structure of Ca 2 FeReO 6 , whereas cubic CaCu 3 Fe 2 Re 2 O 12 is more isotropic. A few double perovskites have higher Curie temperatures than CaCu 3 Fe 2 Re 2 O 12 , for example 600 K in Sr 2 CrReO 6 and 725 K in Sr 2 CrOsO 6 , but these materials have far smaller saturated magnetizations, of 1.9 and 1.8 μ B (double f.u.) −1 , respectively [22] , [50] , [51] . Hence, CaCu 3 Fe 2 Re 2 O 12 is notable among magnetic oxides in offering both a high T c and a large saturated magnetization. Electronic structure and magnetotransport properties of CaCu 3 Fe 2 Re 2 O 12 Spin-polarized electronic structure calculations converge to the observed ferrimagnetic CaCu 2+ (↑) 3 Fe 3+ (↑) 2 Re 5+ (↓) 2 O 12 ground state irrespective of the initial spin structure, showing that this ground state is very stable. The total magnetic moment is 9.0 μ B f.u. −1 and the calculated magnetic moments inside the muffin-tin spheres for Cu, Fe and Re are respectively 0.39, 4.03 and −0.72 μ B , which are slightly reduced from ideal 2 S values due to strong hybridization with O 2 p orbitals. An important prediction from the calculations is that CaCu 3 Fe 2 Re 2 O 12 is half-metallic with fully spin-polarized conduction electrons, as shown in Fig. 6 . The electronic band structure has a large gap in the up(majority)-spin bands and only down(minority)-spin bands of mainly Re 5 d hybridized with O 2 p states cross the Fermi level ( E F ). In contrast, Ca 2 FeReO 6 is predicted to be an insulator with gaps at E F for both majority-spin and minority-spin bands and does not show metallic conductivity [47] , [52] . 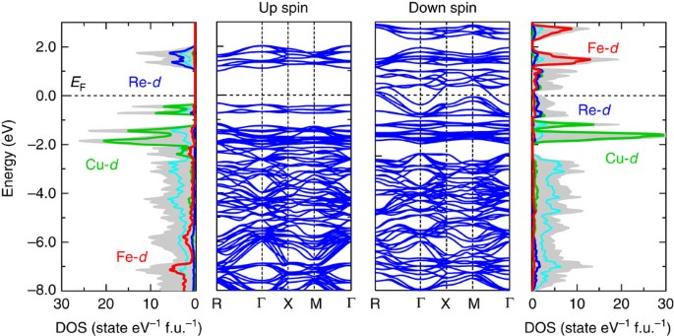Figure 6: Electronic structure of ferrimagnetic CaCu3Fe2Re2O12. Calculated density of states (DOS) and band structures for up-spin and down-spin electrons. Total DOS (shaded regions) and partial DOS of Cu (green curves), Fe (red curves), Re (blue curves) and O (light blue curves) are shown. Only the down(minority)-spin bands cross the Fermi level (EF) as there is a gap in the up(majority)-spin bands. The calculation reproduces the CaCu2+(3d9,S=1/2: ↑)3Fe3+(3d5,S=5/2: ↑)2Re5+(5d2,S=1: ↓)2O12ferrimagnetic spin structure well. Figure 6: Electronic structure of ferrimagnetic CaCu 3 Fe 2 Re 2 O 12 . Calculated density of states (DOS) and band structures for up-spin and down-spin electrons. Total DOS (shaded regions) and partial DOS of Cu (green curves), Fe (red curves), Re (blue curves) and O (light blue curves) are shown. Only the down(minority)-spin bands cross the Fermi level ( E F ) as there is a gap in the up(majority)-spin bands. The calculation reproduces the CaCu 2+ (3 d 9 , S =1/2: ↑) 3 Fe 3+ (3 d 5 , S =5/2: ↑) 2 Re 5+ (5 d 2 , S =1: ↓) 2 O 12 ferrimagnetic spin structure well. Full size image Resistivity and magnetoresistance measurements on a ceramic pellet of CaCu 3 Fe 2 Re 2 O 12 are shown in Fig. 7 . The resistivity is near 10 mΩ cm at room temperature and the observed slight increase on cooling (inset of Fig. 7a ) would correspond to an unrealistically small gap energy of <1 meV if CaCu 3 Fe 2 Re 2 O 12 was semiconducting. This suggests that grain boundary resistances mask the underlying metallic conductivity. The observed conducting behaviour of CaCu 3 Fe 2 Re 2 O 12 is different from the insulating behaviour of CaCu 3 Fe 2 Sb 2 O 12 (ref. 35 ) and the semiconductivity of charge-disproportionated CaCu 3 Fe 4 O 12 (ref. 38 ). Spin-polarized conduction is revealed by the decrease in low-temperature resistivity of the sample under magnetic fields with a sharp low-field magnetoresistance contribution at magnetic fields <3 kOe. This is indicative of spin-dependent tunnelling of spin-polarized conduction electrons through grain or domain boundaries [53] . Close inspection shows that the hysteresis in low-field magnetoresistance slightly differs from that in the magnetization, as the peak-to-peak magnetoresistance separation does not coincide with the coercive field value ( Fig. 7b ). The behaviour is similar to that observed in half-metallic Sr 2 FeMoO 6 and suggests a spin-valve-type magnetoresistance due to the intergrain tunnelling of spin-polarized conduction carriers [54] . Although the observed magnetoresistance ratio of our ceramic CaCu 3 Fe 2 Re 2 O 12 sample is small, most likely due to the slight Fe/Re antisite disorder and the effect of small (≈140 nm) B-cation-ordered domains as discussed for Sr 2 FeMoO 6 (ref. 26 ), the low-field magnetoresistance indicates that conduction electrons are spin-polarized in the quadruple perovskite CaCu 3 Fe 2 Re 2 O 12 . 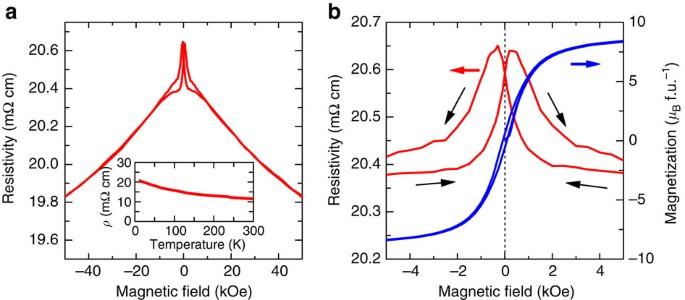Figure 7: Transport properties of CaCu3Fe2Re2O12. (a) Magnetic field dependence of resistivity measured at 10 K with external fields from −50 to 50 kOe. Inset shows temperature dependence of zero-field resistivity. (b) A magnified view of the field dependence of resistivity and magnetization on cycling. The observed low-field spin-valve-type magnetoresistance reveals intergrain tunnelling of spin-polarized conduction carriers. Figure 7: Transport properties of CaCu 3 Fe 2 Re 2 O 12 . ( a ) Magnetic field dependence of resistivity measured at 10 K with external fields from −50 to 50 kOe. Inset shows temperature dependence of zero-field resistivity. ( b ) A magnified view of the field dependence of resistivity and magnetization on cycling. The observed low-field spin-valve-type magnetoresistance reveals intergrain tunnelling of spin-polarized conduction carriers. Full size image The new quadruple perovskite CaCu 3 Fe 2 Re 2 O 12 synthesized by high-pressure and -temperature synthesis is cation ordered at both A and B sites, and has a cubic structure with formal charge distribution Ca 2+ Cu 2+ 3 Fe 3+ 2 Re 5+ 2 O 12 . Strong antiferromagnetic coupling of Re 5+ spins to those of Cu 2+ and Fe 3+ results in ferrimagnetic CaCu 2+ (↑) 3 Fe 3+ (↑) 2 Re 5+ (↓) 2 O 12 order with a high transition temperature (560 K) and a large magnetization (8.7 μ B f.u. −1 ). XAS-MCD and neutron diffraction measurements confirm the ferrimagnetic spin structure. Electronic structure calculations predict that the ferrimagnetic ground state is half-metallic with only minority-spin bands crossing the Fermi level, producing highly spin-polarized conduction electrons. Resistivity measurements confirm spin-polarized conduction and a low-field spin-valve-type magnetoresistance is evident, although further optimization to suppress Fe/Re disorder fully is needed. The combination of a high magnetic ordering temperature and large magnetization, in comparison to double-perovskite analogues, and spin-polarized conductivity demonstrates that the introduction of further magnetic cations that can participate in a 1:3 order at the A sites is a good strategy for discovery of a new family of spintronic quadruple perovskite oxide materials. Sample preparation A polycrystalline sample of CaCu 3 Fe 2 Re 2 O 12 was prepared by a solid-state reaction at a high temperature and high pressure. Stoichiometric amounts of Ca 2 Fe 2 O 5 , CuO, Cu 2 O, ReO 3 and Fe 2 O 3 were well mixed and the mixture was sealed in a platinum capsule. The assembled sample cell was placed in a DIA-type cubic anvil high-pressure apparatus and treated at 10 GPa and 1400 K for an hour. Crystal structure analysis A SXRD experiment was carried out for phase identification and crystal structure analysis. The room-temperature SXRD pattern obtained with a wavelength of 0.498856 Å was recorded on the image plate of a large Debye–Scherrer camera installed at beamline BL02B2 in SPring-8. The powder sample was placed in a 0.1 mm glass capillary tube to minimize absorption and rotated during the measurement. The obtained data were analysed with the Rietveld method by using the TOPAS software package. Magnetic and transport property measurements Magnetic properties were measured with a commercial magnetometer (Quantum Design Magnetic Properties Measurement System). Temperature dependence of the magnetic susceptibility was measured at 5–700 K in an external magnetic field of 10 kOe. Field dependence of the magnetization was measured at several temperatures under fields ranging from −50 to 50 kOe. X-ray MCD spectra were obtained by a total electron yield method from X-ray absorption experiments conducted at beamline BL25SU in SPring-8. The powder sample was pasted uniformly on a sample holder by using carbon tape. The spectra at 15 K were obtained using parallel ( I + ) and antiparallel ( I - ) photon spins along the magnetization direction of the sample, to which a static magnetic field of 19 kOe was applied. The MCD intensity was defined as the difference between the two absorption spectra ( I MCD = I - − I + ). Transport properties of the sample were measured in a conventional four-probe configuration. The temperature dependence of the resistivity and magnetoresistance were measured under magnetic fields ranging from −50 to 50 kOe. Electronic structure calculation The electronic structure of CaCu 3 Fe 2 Re 2 O 12 was calculated by full-potential linearized augmented plane-wave first-principle calculations with the WIEN2k code. The lattice constant and atomic position parameters obtained from the structural refinement were used for the calculation. The full-potential linearized augmented plane-wave sphere radii for Ca, Cu, Fe, Re and O were respectively 2.0, 1.9, 1.9, 1.9 and 1.60 a.u. An effective U eff (= U−J ) of 4 eV was introduced for B-site Fe and B′-site Re. Self-consistency was carried out on 1000 k -point meshes in the whole Brillouin zone. Neutron powder diffraction for magnetic structure analysis Neutron powder diffraction from a ~0.8 g polycrystalline CaCu 3 Fe 2 Re 2 O 12 powder sample in a 5-mm-diameter vanadium was carried out using the D20 diffractometer at the Institut Laue-Langevin (ILL), Grenoble, France. The diffraction patterns were collected with a neutron wavelength of 2.4194 Å. The crystal and magnetic structures of data collected at 5 K were fitted by the Rietveld method using the General Structure Analysis System software package and the obtained results are shown in Supplementary Fig. S1 and Supplementary Table S1 . Fe/Re inversion was not refined as these two elements have very similar nuclear scattering factors; b(Fe)=9.5 fm and b(Re)=9.2 fm. How to cite this article: Chen, W.-t. et al. A half-metallic A- and B-site-ordered quadruple perovskite oxide CaCu 3 Fe 2 Re 2 O 12 with large magnetization and a high transition temperature. Nat. Commun. 5:3909 doi: 10.1038/ncomms4909 (2014).